Diffusion driven layer-by-layer assembly of graphene oxide nanosheets into porous three-dimensional macrostructures Despite recent progress in preparing numerous types of nanosheets, it remains a difficult challenge to assemble the tiny building blocks into functional macroscale architectures suitable for practical applications. Here we introduce a diffusion driven layer-by-layer assembly process and demonstrate its application for the construction of graphene oxide sheets into various three-dimensional structures. This process involves complexation of the negatively charged graphene oxide sheets and positively charged branched polyethylenimine at a given interface. We find that the diffusion of branched polyethylenimine molecules allows the complex to continuously grow into foam-like frameworks with tunable porosities. Furthermore, the assembly process is quite robust and can be utilized in various configurations such as to create free-standing architectures with tailored shapes or patterned films on a substrate. With such useful features, we believe that this technique may serve as a valuable tool for the assembly of nanomaterials. Significant development in both physical and chemical exfoliation techniques during the past several years has allowed the production of nanosheets from a wide range of layered materials, including graphite, transitional metal dichalcogenides, oxides, and tertiary carbides and nitrides [1] , [2] , [3] , [4] , [5] , [6] , [7] . The nanosheets are sought after for various applications such as ultracapacitors, battery electrodes, filtration membranes and sensors [8] , [9] , [10] , [11] , [12] , [13] , [14] , [15] . However, in order to integrate the nanosheets into such real-life devices, it is often necessary to construct them into suitable two-dimensional (2D) or three-dimensional (3D) macrostructures. As a result, developing methods to assemble the nanosheets with good control and efficiency becomes a critical challenge. Forming nanosheets into thin-film structures can be generally done with good precision and simplicity using well-established strategies such as spin-coating [16] , filtration [17] , [18] , layer-by-layer (LbL) assembly [19] , [20] , and Langmuir–Blodgettry [21] , [22] . On the other hand, creating thicker structures has been a more difficult task. An important characteristic of nanosheets is its high-surface area. However, the nanosheets can easily aggregate during assembly, leading to significantly decreased surface area and thus diminished material properties. Therefore, the main question becomes how to construct the nanosheets into 3D macrostructures while suppressing aggregation. Few promising directions have been explored to address this issue, especially using graphene oxide (GO) nanosheets. For example, several researchers have demonstrated hydrothermal treatment of GO suspension as a versatile method to produce various types of porous graphene frameworks [23] , [24] , [25] , [26] . Vermant and colleagues [27] reported the preparation of GO frameworks from bi-continuous emulsions stabilized by the nanosheets. Niu et al. [28] introduced a leavening process, showing that tightly packed GO films can be inflated into a foam-like structure by the gas evolution during reduction of GO. Inclusion of spacers between the GO layers, such as nanoparticles or polymer beads, has also been widely investigated [11] , [29] , [30] . Such developments have opened new ways to obtain diverse graphene-based macrostructures that exhibit favourable properties for applications such as sensors and energy storage. On the other hand, it remains a difficult challenge to direct the construction of nanosheets with good control over the shape of the assembled structure. For instance, moulding the GO into tailored forms, such as sphere, cube and fibre, is not as straightforward to achieve using conventional methods and generally requires elaborate experimental setups. Another example would be growing thick graphene films at selected pre-patterned area of a given substrate, which is potentially important for device fabrication purposes. Furthermore, the aforementioned assembly techniques mostly rely on the inherent characteristics of GO, and therefore is unlikely to be easily applicable to the assembly of different types of nanomaterials. We previously reported a strategy for directing the assembly of nanosheets into various macrostructures through interfacial polyionic complexation [31] . A key point of the study was that nanosheets often behave as charged macromolecules and therefore can form a stable complex with oppositely charged polyelectrolytes. Such characteristic was explored using chitosan, a positively charged biopolymer, that readily interacted with nanosheets that have negative surface charges such as GO, WS 2 and MoS 2 . We found that the complexation could be confined at liquid–liquid or air–liquid interfaces, which allowed control over the nanosheet assembly into forms such as films, fibres and capsules. These results suggest that interfacial polyionic complexation could be a useful tool for guiding the assembly of nanosheets in a simple way. At the same time, we noticed that the nanosheet/chitosan complex typically stops growing after reaching a thickness of few tens of nanometres, which is owing to the layer acting as a barrier that blocks further reaction. This has been a limiting factor in tuning the assembly process, especially for creating thicker macrostructures. Herein, we report a completely different assembly behavior that was observed during the complexation between GO and branched polyethyleneimine (b-PEI). In contrast to the case of chitosan, b-PEI is able to diffuse through the GO/b-PEI complex formed at the interface, which allows the layer to grow in a continuous fashion into 3D structures with thickness reaching millimetre ranges. Furthermore, the assembled structures display a foam-like porous feature. The GO/b-PEI structure formation occurs in a way that resembles a LbL assembly. On the other hand, rather than requiring multiple deposition steps, the assembly is driven by diffusion of b-PEI and therefore, once initiated, can progress without additional external force or stimuli. Based on such observations, we propose a new type of assembly method, namely ‘diffusion driven layer-by-layer (dd-LbL) assembly’. This process is quite robust and can be utilized in various ways to create a wide range of macrostructures. For example, in this report, we demonstrate the assembly of GO nanosheets into porous frameworks with adjustable porosity, growth of patterned multilayered films on solid and flexible substrates, and preparation of free-standing 3D structures which shape can be controlled through the use of templates. With such set of useful capabilities, we strongly believe that this ‘dd-LbL assembly’ will be able to serve as a versatile technique for constructing nanosheets into diverse 3D macrostructures. dd-LbL assembly of GO and b-PEI Polyethylenimine (PEI) is a positively charged polyelectrolyte that contains amine functional groups. It is used in various industrial applications such as paper production, detergent and water treatments. PEI is commercially available in both linear and branched forms. However, owing to limited solubility of linear PEI in water at room temperature, we focus mainly on branched PEI for this study. To examine the interaction of b-PEI and GO at a liquid–liquid interface, droplets of a b-PEI solution ( M w =750,000, M n =60,000, 25 wt.% in water, ~12 μl) were added to a GO suspension (8 mg ml −1 in dimethylformamide (DMF):water=9:1 mixture) and left for several hours ( Fig. 1a ). This induced complexation of GO and b-PEI at the droplet surface, which was demonstrated by the formation of a dark brown layer surrounding the droplet ( Fig. 1b ). Interestingly, the size of the sphere became significantly larger compared with the initial b-PEI droplet, showing a diameter increase from 2.8 mm to ~6.5 mm. Furthermore, the layer was sufficiently stable enough such that the wet structure could preserve its spherical shape even after being left in air or manipulated by a pair of tweezers. For simplicity, we will call this product GO/b-PEI bead. Cutting the bead with a razor blade revealed that the shell thickness was in the range of several millimetres ( Fig. 1c ). Further in-depth structure of the GO/b-PEI complex layer was investigated by scanning electron microscopy (SEM; Fig. 1d–f ). For sample preparation, the bead was dried by freeze-drying to minimize structural changes. SEM images show that the GO nanosheets formed a highly porous network, suggesting that the initial wet structure contained a large volume of water. In addition, the nanosheets are mostly arranged in a layered configuration despite the large voids, forming an onion-like architecture composed of numerous concentric shells. It should be noted that drying the sample in an oven or in air leads to substantial structural changes, likely owing to surface tension of the water pulling the GO sheets together during evaporation. In fact, such phenomena could be utilized as a way to adjust the porosity of the assembled structure, as will be discussed in more detail below. 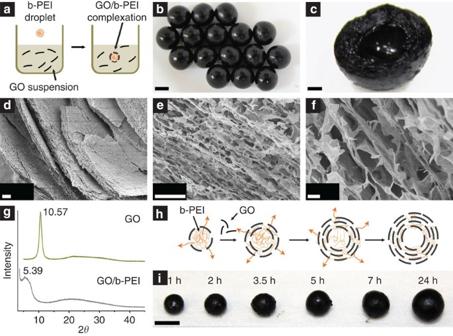Figure 1: Diffusion driven layer-by-layer assembly of GO. (a) Schematic representation of an experimental setup. When droplets of branched polyethylenimine (b-PEI) solution are added to a GO suspension, complexation between b-PEI and GO occurs at the droplet surface. This results in the formation of stable bead-like structures (b). (c) Cross-section of a bead shows that the layer of GO/b-PEI complex is a few millimetres thick. Furthermore, from SEM images (d–f), we find the nanosheets form a layered and porous network. (g) XRD analysis reveals an increase of interlayer distance in GO, suggesting that b-PEI is serving as a binder between the nanosheets. (h) Proposed assembly mechanism. Key point is the ability of b-PEI to diffuse through the GO/b-PEI complex, which allows continuous growth of the layer into thick macrostructures without any additional treatments. (i) Longer reaction time produces larger beads, supporting the hypothesis that the assembly is driven by the diffusion of b-PEI. Scale bars, (b) 5 mm, (c) 1 mm, (d) 100 μm, (e) 10 μm, (f) 1 μm and (i) 5 mm. Figure 1: Diffusion driven layer-by-layer assembly of GO. ( a ) Schematic representation of an experimental setup. When droplets of branched polyethylenimine (b-PEI) solution are added to a GO suspension, complexation between b-PEI and GO occurs at the droplet surface. This results in the formation of stable bead-like structures ( b ). ( c ) Cross-section of a bead shows that the layer of GO/b-PEI complex is a few millimetres thick. Furthermore, from SEM images ( d – f ), we find the nanosheets form a layered and porous network. ( g ) XRD analysis reveals an increase of interlayer distance in GO, suggesting that b-PEI is serving as a binder between the nanosheets. ( h ) Proposed assembly mechanism. Key point is the ability of b-PEI to diffuse through the GO/b-PEI complex, which allows continuous growth of the layer into thick macrostructures without any additional treatments. ( i ) Longer reaction time produces larger beads, supporting the hypothesis that the assembly is driven by the diffusion of b-PEI. Scale bars, ( b ) 5 mm, ( c ) 1 mm, ( d ) 100 μm, ( e ) 10 μm, ( f ) 1 μm and ( i ) 5 mm. Full size image X-ray diffraction (XRD) analysis of the GO/b-PEI bead shows a peak at a smaller angle (2 θ =5.39°, d =1.64 nm) compared with a solid sample of unmodified GO (2 θ =10.57°, d =0.84 nm) ( Fig. 1g and Supplementary Fig. 1 ). Such increase in interlayer spacing suggests that b-PEI becomes incorporated between the GO layers during the assembly process. Fourier transform infrared (FT-IR) spectrum of GO shows peaks at 1,730 cm −1 from C=O (carbonyl) stretching and 1,626 cm −1 from C=C (aromatic) stretching ( Supplementary Fig. 2 ). However, the carbonyl peak becomes no longer noticeable after complexation with b-PEI. In addition, characteristic peak from the amine group of b-PEI (1,659 cm −1 ) is also not observed from the complex ( Supplementary Fig. 2 ). This suggests that the carbonyl group of GO and amine group of b-PEI are strongly interacting with each other, leading to peak shifts overlapping with the broad C=C peak. Based on such observations, we propose the following mechanism for the bead formation ( Fig. 1h ). As the b-PEI droplet is immersed into a GO suspension, complexation between the polyelectrolyte and nanosheets occurs at the interface due to electrostatic interactions. This produces a thin complex layer encapsulating the droplet, the outer surface of which is dominated by negatively charged GO. Despite such layer formation, b-PEI is able to penetrate the barrier and continuously diffuse out through the interspace between GO sheets, most likely driven by osmotic pressure. Some of the diffused b-PEI attaches to the negatively charged outer surface, leading to additional deposition of GO onto the shell. At the same time, this leads to depletion of GO in the vicinity, which allows the other portion of b-PEI to diffuse further out and create a new interface apart from the initial complexation layer, resulting in the large void between layers. This cycle of complexation–diffusion–complexation allows continuous formation of GO shells around the b-PEI droplet, eventually building up the layered and porous 3D macrostructures shown in Fig. 1 . It should be noted that the reactants are continuously consumed as the assembly progresses. This is likely to lead to decreased frequency of complexation and thus slower growth of the assembled structure with time. Indeed, we observe that although the size of the GO/b-PEI beads does increase with longer reaction time, not much change is noticed after 24 h ( Fig. 1i ). Our proposed assembly model is further supported by quantitative analysis on the GO/b-PEI layer growth ( Supplementary Fig. 3 ). It can be noticed that while the thickness of the shell increases with time, size of the inner hollow core remains mostly unchanged from the initial b-PEI solution droplet. This matches well with our hypothesis that the GO/b-PEI complexation first occurs at the surface of the droplet (that is, interface between the two solutions) and then grows towards the direction of the GO suspension owing to b-PEI molecules travelling across the interface. Interfacial complexation induced within a transparent tube also confirms that the reaction mostly occurs on the GO side ( Supplementary Fig. 4 ). Decrease in growth rate of the GO/b-PEI layer with time is also clearly observed; this indicates that although the assembly is driven by the diffusion of b-PEI, other factors such as depletion of the reactants can influence the growth of the assembled structure. Similar diffusion-induced development of complex layer has also been observed during interactions between oppositely charged small molecules at liquid–liquid interfaces [32] , [33] , [34] ; however, the formation of a porous multilayered structure shown in Fig. 1 is quite unique, which we attribute to the relatively large size and highly anisotropic shape of the GO sheets. In a previous study, we have explored the interaction between GO and chitosan under similar experimental setups [31] . The formation of GO/chitosan complex layer was still observed at the droplet surface; however, the layer thickness was very thin and did not grow beyond 100 nm. Results in Fig. 1 suggest that a critical factor for the continuous assembly of nanosheets to occur is whether the polyelectrolyte can penetrate the initial complexation layer. Although we do not yet fully understand what requisites need to be satisfied for this, comparison between chitosan and b-PEI provides some insights. We believe that two factors may be of importance, which are (1) strength of the GO/polyelectrolyte and polyelectrolyte/polyelectrolyte interaction and (2) solubility of the polyelectrolyte. Chitosan is a linear polysaccharide that contains large number of hydroxyl and amine groups. Therefore, it can form strong hydrogen bonding not only with GO but also with other chitosan molecules. This is likely to result in formation of a tightly bound complexation layer. On the other hand, the interaction between branched polymer chains such as b-PEI is generally weaker than that of linear polymers due to steric hindrance. In addition, b-PEI only contains amine groups and therefore do not form hydrogen bonding with other b-PEI molecules. Therefore, we can presume that the complexation layer of b-PEI and GO to be more loosely bound, which allows b-PEI to diffuse through the barrier. Similar considerations play a role in regard to the electrolyte solubility. Chitosan solution becomes viscous and gel-like even at comparatively low concentrations owing to strong interactions and entanglement between the polymer chains. As a result, the highest concentration that we could test was 2 wt. %. On the other hand, b-PEI solutions can easily be prepared in high concentrations owing to relatively weak intermolecular interactions. For example, results in Fig. 1 were produced using a 25 wt. % solution. Higher polymer concentration can be translated into stronger osmotic pressure and thus faster diffusion. Indeed, when a 10 wt. % b-PEI solution was used, the size of GO/b-PEI bead was noticeably smaller, and below that concentration the complexation layer did not form properly ( Supplementary Fig. 5 ). This suggests that higher concentrations of polyelectrolyte solution may be another important requisite for the multilayered assembly to occur. However, there are several other factors that could influence the behavior of polyelectrolytes such as molecular weight, solvent and pH, and further studies are needed to more accurately elucidate the assembly mechanism. The process of building up multilayered structures through alternating layers of oppositely charged materials as depicted in Fig. 1h shares some similarities with conventional LbL assembly. At the same time, rather than going through multiple deposition cycles, the assembly is driven by diffusion and as a result, once initiated, can progress in a continuous fashion without additional treatments. Therefore, we use a new term ‘dd-LbL assembly’ to describe this unique process. Despite its simplicity, this assembly technique is quite versatile and can be utilized in various ways to construct a wide range of graphene-based superstructures with adjustable properties and shapes, as will be discussed throughout the rest of this report. Properties of the assembled GO/b-PEI structures An interesting characteristic of the structures produced by dd-LbL assembly is that they exhibit foam-like porous features as displayed in the SEM images shown in Fig. 1 . The porosity and stability of the assembled products can be further demonstrated by a simple oil-absorbing experiment. When a freeze-dried bead was placed on top of a pool of pump oil, it rapidly absorbed the oil up to 35 times its own mass ( Fig. 2a ). The beads could be recycled by immersing them into hexane to drain the absorbed oil. After the sample dried, it returned back to its initial weight while the spherical structure was well preserved ( Fig. 2a , bottom right). There was no significant change in the oil-absorbing capacity even after several cycles, which illustrates the stability of the porous structure ( Fig. 2b ). In addition, the beads showed similar absorbing efficiency with other types of solvents such as toluene, olive oil and chloroform (30, 28 and 34 times its own mass, respectively; Fig. 2c ). 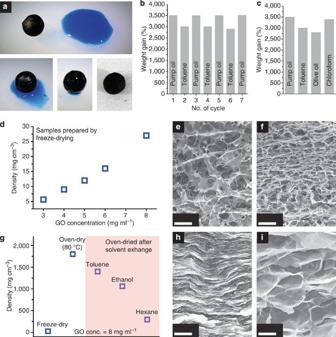Figure 2: Porosity of the GO/b-PEI beads produced by dd-LbL assembly. (a) When placed on top of a pool of pump oil, the GO/b-PEI bead rapidly absorbs the oil owing to its porous nature. The bead can be recycled by immersing it in hexane to drain the absorbed oil and then drying it under ambient conditions. (b) Oil absorption experiment alternating between pump oil and toluene. Even after several cycles, there is no noticeable change in the absorption efficiency, demonstrating its structural stability. (c) Similar absorption efficiency is observed for other nonpolar solvents. (d) Density of the beads prepared from GO suspensions of varying concentrations. Lower GO concentrations result in beads with lower densities, or in other words, higher porosity. This is confirmed by SEM, withe,fdisplaying samples prepared with concentrations of 3 and 5 mg ml−1, respectively. These samples were dried by freeze-drying. (g) However, using different drying method can also influence the porosity. For example, when dried in an 80 °C oven, the surface tension of water pulls the GO sheets together into a densely packed multilayered film (h). Intermediate densities can also be achieved by exchanging the water to solvents with lower surface tension, such as hexane, before drying (i). Scale bars, (e,f) 10 μm and (h,i) 1 μm. Figure 2: Porosity of the GO/b-PEI beads produced by dd-LbL assembly. ( a ) When placed on top of a pool of pump oil, the GO/b-PEI bead rapidly absorbs the oil owing to its porous nature. The bead can be recycled by immersing it in hexane to drain the absorbed oil and then drying it under ambient conditions. ( b ) Oil absorption experiment alternating between pump oil and toluene. Even after several cycles, there is no noticeable change in the absorption efficiency, demonstrating its structural stability. ( c ) Similar absorption efficiency is observed for other nonpolar solvents. ( d ) Density of the beads prepared from GO suspensions of varying concentrations. Lower GO concentrations result in beads with lower densities, or in other words, higher porosity. This is confirmed by SEM, with e , f displaying samples prepared with concentrations of 3 and 5 mg ml −1 , respectively. These samples were dried by freeze-drying. ( g ) However, using different drying method can also influence the porosity. For example, when dried in an 80 °C oven, the surface tension of water pulls the GO sheets together into a densely packed multilayered film ( h ). Intermediate densities can also be achieved by exchanging the water to solvents with lower surface tension, such as hexane, before drying ( i ). Scale bars, ( e , f ) 10 μm and ( h , i ) 1 μm. Full size image Owing to its porous nature, the assembled GO/b-PEI structures are quite light. For instance, the product shown in Fig. 1 has a density of ~27 mg cm −3 , similar with that of ‘GO foams’ produced through a leaving process as reported by Niu et al. [28] At the same time, the sample porosity can be further tuned with simple modifications to the experimental conditions. One such method is to adjust the GO concentration. In general, lower concentrations lead to structures with lower densities or, in other words, higher porosity, as shown in Fig. 2d . The structural differences can be also confirmed by SEM, with samples prepared at GO concentrations of 3 mg ml −1 ( Fig. 2e ) and 5 mg ml −1 ( Fig. 2f ), clearly exhibiting looser networks compared with that prepared at 8 mg ml −1 ( Fig. 1 ). Such changes in porosity can be well explained by our proposed assembly mechanism. Even after b-PEI diffuses into the GO suspension, the two components need to get into contact for the complexation to occur. At lower GO concentrations, b-PEI is likely to diffuse longer distances before eventually interacting with the nanosheets to form a stable complex, thereby leading to a more loosely packed structure and larger macroscopic pores. This is in good agreement with the observed results. For the same reasons, we can also expect the overall size of the assembled structure to be larger at lower GO concentrations, which is indeed the case ( Supplementary Fig. 6 ). The lowest concentration we were able to obtain a stable structure from was 3 mg ml −1 , which produced a sample with density of 5.6 mg cm −3 . This value is comparable to those of ultralight graphene frameworks produced by hydrothermal treatment of GO [25] or chemical vapour deposition on metal foams [35] . It should be noted that the low density, highly porous structures discussed above were obtained when the samples were dried by freeze-drying. During this process, not much change was noticed in the overall size and shape of the product. On the other hand, even with samples prepared under identical experimental conditions, using different drying procedures can lead to substantial structural changes. For example, the GO/b-PEI layer, the thickness of which was~2 mm in its initial wet state ( Fig. 1c ) shrinks into a thin layer of ~50 μm when dried in an oven at 80 °C ( Supplementary Fig. 7 ). SEM confirms the formation of a dense, tightly packed multilayer film ( Fig. 2h ), which can be explained by the surface tension of water pulling the GO sheets together during evaporation. In contrast, freeze-drying the sample minimizes such effect and helps preserve the porous structure. Interestingly, such phenomena can be utilized as another method to adjust the sample porosity. By first exchanging the solvent within the GO/b-PEI bead to another solvent with lower surface tension, such as ethanol, hexane and toluene, and then drying in the oven, we find that it is possible to produce intermediate structures that are lighter than the packed multilayer but are still denser than the freeze-dried samples ( Fig. 2g,i ). Although we have discussed only two factors here, namely GO concentration and the drying method, adjusting other parameters such as b-PEI concentration or solvents may also lead to similar behaviours. One important question regarding the obtained products is how the presence of b-PEI may affect the properties of GO. In particular, as reduced GO (r-GO) is actively pursued for applications such as ultracapacitors, battery electrodes and sensors, the conductivity and stability of the assembled GO/b-PEI structure after reduction is of strong interest. To address this question, we first examine the content of b-PEI within the product through thermogravimetric analysis (TGA) and X-ray photoelectron spectroscopy (XPS). Samples produced at GO concentration of 8 mg ml −1 , identical to those in Fig. 1 , were used for the analysis. TGA result ( Fig. 3a ) displays two distinct steps, the first corresponding to deoxygenation of GO and the second to decomposition of b-PEI. The deoxygenation of GO starts at a lower temperature compared with pristine GO; this may be possibly owing to the interaction of the oxygen-based functional groups of GO with the amine group of b-PEI. From the weight loss, we estimate the amount of b-PEI within the sample to be ~35% in mass. This value was also confirmed by elemental analysis from XPS ( Supplementary Fig. 8 ). A point to note from TGA is that b-PEI almost fully decomposes at temperatures >400 °C, leaving only a small residue of <15% of its original mass. Despite such reactions, the samples are surprisingly stable. For instance, Fig. 3b displays a GO/b-PEI bead after thermal treatment at 450 °C under nitrogen atmosphere for 30 min. Not much change is noticed to the overall size and shape of the bead and the microscopic porous network is also well preserved. At the same time, the decomposition of b-PEI leads to enhanced conductivity of the r-GO structure, as shown below. 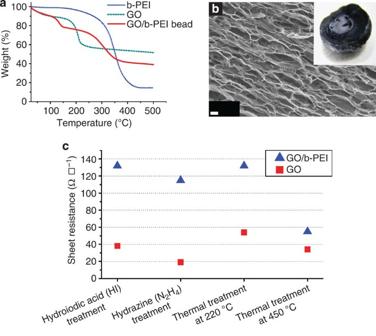Figure 3: Properties of the assembled GO/b-PEI structures. (a) From TGA, the composition of b-PEI within a GO bead can be estimated to be ~35% in mass. At the same time, the result implies that significant portion of b-PEI becomes decomposed at temperatures >400 °C. (b) Despite such reactions, the samples show good thermal stability. Image shows a GO/b-PEI bead after thermal treatment at 450 °C. Not much change is noticed in both the porous framework and overall structure (inset). (c) The assembled GO/b-PEI structures can be reduced using various methods, after which the sheet resistances become slightly higher, but comparable to pure GO samples reduced under identical conditions. In particular, the samples that were thermally treated at 450 °C show improved conductivity, which is likely owing to decomposition of b-PEI. Scale bar, 1μm (b). Figure 3: Properties of the assembled GO/b-PEI structures. ( a ) From TGA, the composition of b-PEI within a GO bead can be estimated to be ~35% in mass. At the same time, the result implies that significant portion of b-PEI becomes decomposed at temperatures >400 °C. ( b ) Despite such reactions, the samples show good thermal stability. Image shows a GO/b-PEI bead after thermal treatment at 450 °C. Not much change is noticed in both the porous framework and overall structure (inset). ( c ) The assembled GO/b-PEI structures can be reduced using various methods, after which the sheet resistances become slightly higher, but comparable to pure GO samples reduced under identical conditions. In particular, the samples that were thermally treated at 450 °C show improved conductivity, which is likely owing to decomposition of b-PEI. Scale bar, 1μm ( b ). Full size image To examine the influence of b-PEI to conductivity, we reduced the obtained products in four different ways, namely hydroiodic acid (HI) treatment, hydrazine (N 2 H 4 ) treatment and thermal treatment at 220 and 450 °C, and measured their sheet resistances using a four-probe setup (Jandel HM21 model). For this experiment, the GO/b-PEI samples were prepared in film forms rather than beads to avoid the difficulty of measuring round surfaces. Films can be easily produced with small modifications to the experimental setups as will be discussed in the next section. Structure of the samples was well preserved even after reduction. Furthermore, all samples showed good recovery of conductivity, with the resistances slightly higher but comparable with pure GO films reduced under identical conditions ( Fig. 3c ). In particular, with thermal reduction at 450 °C, the resistance difference between GO/b-PEI and pure GO became quite small, which can be attributed to the decomposition of b-PEI. These results suggest that although the presence of b-PEI may lead to slightly decreased conductivity of the r-GO, such influence can be minimized by removing the polyelectrolyte through thermal treatments. Forming GO/b-PEI film on solid/flexible substrates Up to this point, we have mainly examined the dd-LbL assembly using the formation of bead structures by complexation of GO and b-PEI on a liquid droplet surface. However, with simple modifications to the experimental configuration, it is possible to construct a much wider range of 3D architectures. For example, instead of adding a droplet of b-PEI solution directly into a GO suspension, one can first apply it on a glass substrate as shown in Fig. 4a . Note that green dye was added to the solution for easier visualization. When the glass slide is immersed in a GO suspension (8 mg ml −1 ) for several hours, a thick film forms over the area where the b-PEI droplet was originally applied to ( Fig. 4b ). Based on previous discussions, it is reasonable to expect that such film formation is also driven by diffusion of b-PEI from the deposited droplet or, in other words, through dd-LbL assembly. Indeed, the properties and microstructures of such GO/b-PEI films show strong resemblance with those of the beads. When freeze-dried, the overall shape of the film is well preserved. At the same time, cross-sectional SEM image ( Fig. 4c ) reveals a porous network of GO similar to that observed from the beads ( Fig. 1 ). On the other hand, when dried in an oven, the sample shrinks into a tightly packed multilayered film ( Fig. 4d ) owing to the surface tension of water pulling the GO sheets together as discussed in Fig. 2 . In either case, the nanosheets are mostly oriented parallel to the glass slide. 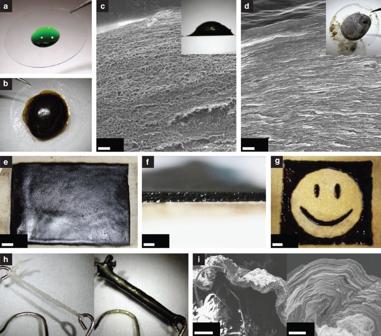Figure 4: Forming GO/b-PEI films on solid and flexible substrates. (a–d) Demonstration on a glass slide. (a) A drop of b-PEI solution is first deposited onto the substrate. (b) When the glass slide is immersed in a GO suspension, a thick film develops over that area. As in the case of beads (Fig. 2), freeze-drying the sample provides a porous foam-like structure (c), whereas oven-drying gives a packed multilayered film (d). (e) Large area (8 cm × 10 cm) film prepared on a filter paper using a similar procedure. Film thickness is fairly uniform throughout the sample (f). The GO/b-PEI film forms only on the area to where b-PEI was applied, which allows patterning of the film into pre-determined shapes (g). (h,i) This assembly can also be performed on non-flat surfaces, such as a thin thread. (i) Cross-sectional SEM confirms the formation of a multilayer coating around the thread. Scale bars, (c) 5 μm, (d) 1 μm, (e) 1 cm, (f) 1 mm, (g) 1 cm, (i, left of panel) 100 μm and (i, right of panel) 10 μm. Figure 4: Forming GO/b-PEI films on solid and flexible substrates. ( a – d ) Demonstration on a glass slide. ( a ) A drop of b-PEI solution is first deposited onto the substrate. ( b ) When the glass slide is immersed in a GO suspension, a thick film develops over that area. As in the case of beads ( Fig. 2 ), freeze-drying the sample provides a porous foam-like structure ( c ), whereas oven-drying gives a packed multilayered film ( d ). ( e ) Large area (8 cm × 10 cm) film prepared on a filter paper using a similar procedure. Film thickness is fairly uniform throughout the sample ( f ). The GO/b-PEI film forms only on the area to where b-PEI was applied, which allows patterning of the film into pre-determined shapes ( g ). ( h , i ) This assembly can also be performed on non-flat surfaces, such as a thin thread. ( i ) Cross-sectional SEM confirms the formation of a multilayer coating around the thread. Scale bars, ( c ) 5 μm, ( d ) 1 μm, ( e ) 1 cm, ( f ) 1 mm, ( g ) 1 cm, ( i , left of panel) 100 μm and ( i , right of panel) 10 μm. Full size image Such preparation of GO/b-PEI film on substrates is quite robust, and we have not yet found much limitation to the type of surface and size of area on which the assembly can be performed. For instance, Fig. 4e displays a film formed on filter paper. To get this, b-PEI solution was first applied to a square area of 8 cm × 10 cm. When the filter paper was immersed in a GO suspension, GO/b-PEI film was developed over the same area. The film thickness is fairly uniform throughout the whole sample, as can be noticed from Fig. 4f . Other than the dimension of the reaction vessel, we have not found much limitation to the size of film that can be produced. The ability to prepare films in such large areas is potentially useful for practical applications. For example, by cutting the film into smaller pieces (2 cm × 2 cm), we were able to easily obtain sufficient number of samples for testing out various reductions methods as presented in Fig. 3c . It should be noted that formation of the GO/b-PEI film is mostly confined to where the b-PEI has been applied, which is natural since the polyelectrolyte is serving as the main element in driving the assembly and keeping the structure intact. In other words, it becomes possible to create patterned films on a given substrate by applying b-PEI only to pre-determined areas, as shown in Fig. 4g . Although this is a simple demonstration, it is not difficult to imagine the preparation of more complex patterns through precise deposition of b-PEI through assistance of conventional techniques such as microfluidics and lithography. Up to now, the patterning of GO on substrates has been mostly limited to single or few layer thin films. The growth of thick multilayered structure, especially with controllable porosity, adds a new dimensionality to the patterning of nanomaterials. Furthermore, this kind of assembly can also be extended to non-flat surfaces. For example, creating a thick GO/b-PEI layer around a thin thread can be easily achieved by first soaking the thread with b-PEI solution and then immersing it in a GO suspension ( Fig. 4h ). As similar to previous results, drying the sample in an oven leads to formation of a packed multilayer film as confirmed by SEM ( Fig. 4i ). These results again demonstrate the versatility of the dd-LbL assembly, which can be performed on surfaces with diverse materials, shapes and sizes, allowing the construction of nanosheets into a wide range of 3D macrostructures. Tailoring the assembled GO/b-PEI structure using templates In addition to methods discussed above, the shape of the assembled products can be also controlled by using templates. 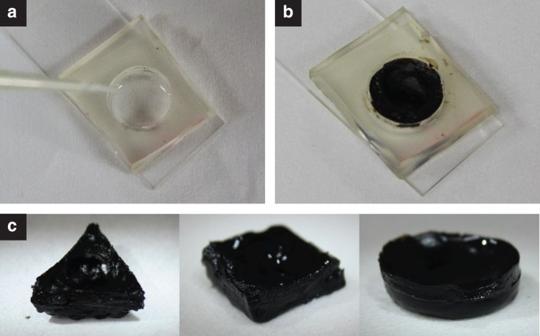Figure 5: Tailoring the assembled GO/b-PEI structure using templates. (a) A polydimethylsiloxane slab with a hole is placed on a glass slide to form a well, to which a small amount of b-PEI solution is applied. (b) When the slide is immersed in a GO suspension, complexation between GO and b-PEI occurs within the confined space and forms a stable macrostructure. (c) The resulting products can be easily released from the template as free-standing pieces. Furthermore, shape of the GO/b-PEI structures closely follows that of the template, allowing the production of diverse forms. Figure 5 shows a simple demonstration of such concept. A polydimethylsiloxane slab with a hole in the middle was placed on a glass slide to form a well. A small amount of b-PEI solution was applied to the bottom of the well ( Fig. 5a ), and then the substrate was immersed in a GO suspension for several hours. Complexation of GO and b-PEI occurred within the well driven by diffusion of the polyelectrolyte ( Fig. 5b ). The GO/b-PEI complex could be easily detached from the polydimethylsiloxane slab and also retained the shape of the template ( Fig. 5c ). Therefore, this provides a simple method to produce free-standing architectures with controllable shapes. Figure 5: Tailoring the assembled GO/b-PEI structure using templates. ( a ) A polydimethylsiloxane slab with a hole is placed on a glass slide to form a well, to which a small amount of b-PEI solution is applied. ( b ) When the slide is immersed in a GO suspension, complexation between GO and b-PEI occurs within the confined space and forms a stable macrostructure. ( c ) The resulting products can be easily released from the template as free-standing pieces. Furthermore, shape of the GO/b-PEI structures closely follows that of the template, allowing the production of diverse forms. Full size image In this report, we introduced a strategy for constructing GO sheets into various 3D macrostructures, namely ‘dd-LbL assembly’. This process is based on polyionic complexation of the negatively charged GO and positively charged b-PEI at an interface. The key point is that the diffusion of b-PEI across the interface allows the complex layer to continuously grow into macroscopic structures without additional external stimuli. Interestingly, the GO/b-PEI complex forms a foam-like porous network, the porosity of which can be tuned from ultralight (5.6 mg cm −3 ) to tightly packed (~1,800 mg cm −3 ) through simple adjustments in experimental condition. Furthermore, the assembly process can be utilized in various configurations such as to create free-standing architectures with tailored shapes or patterned films on a substrate. The simplicity and versatility of this process should be useful in constructing a wide range of 3D graphene-based architectures. At the same time, we believe that this concept of utilizing the diffusion of polyelectrolyte for the assembly of nanosheets into macrostructures should also be applicable to a much wider range of materials. Synthesis of GO GO was synthesized using a modified Hummers method reported earlier [36] . In brief, concentrated H 2 SO 4 (75 ml) was heated to 80 °C in a 500-ml round bottom flask. K 2 S 2 O 8 (15 g) and P 2 O 5 (15 g) were added to the acid and stirred until fully dissolved. Graphite powder (20 g, Bay Carbon Inc. SP-1 grade) was added to the solution and kept at 80 °C for 4.5 h. The mixture was then cooled, diluted with 1.5 l of deionized (DI) water and filtered using filter papers (Whatman, grade no. 3). The collected product was further rinsed with DI water (six times, 1 l each) and dried in air. The powder was then transferred into a 2-l Erlenmeyer flask with concentrated H 2 SO 4 (750 ml) and cooled down to 5 °C using an ice bath. KMnO 4 (100 g) was slowly added to the mixture while stirring. The flask was then transferred to a 35 °C water bath and left for 2 h, and then transferred back into an ice bath. DI water (1 l) was slowly added to the flask while stirring, taking great caution to keep the temperature below 20 °C. The suspension was left for 2 h and then diluted with DI water to a total volume of 4 l. A volume of 80 ml of a 30% H 2 O 2 solution was slowly added to the flask while stirring, forming orange precipitates. The product was filtered using a polytetrafluoroethylene (PTFE) membrane (Millipore, Omnipore membrane, 5.0 μm pores), rinsed with 3.4% HCl solution (1 l at a time, up to a total 6 l), and collected and dried in a desiccator with P 2 O 5 as drying agent. The solid was redispersed in acetone, filtered using a PTFE membrane (Millipore, Fluoropore membrane, 3.0 μm pores), further rinsed with additional acetone (1 l at a time, up to a total 6 l) and dried in ambient conditions. The final product, which is oxidized graphite, was exfoliated into GO by sonicating in water. The exfoliated product was freeze-dried and stored in powder form, which was redispersed in DMF:water (9:1) mixture before use. Formation of GO/b-PEI beads In general, 5–6 droplets of b-PEI solution ( M w =750,000, M n =60,000, 25 wt. % in DI ~12 μl) were added to 10 ml of GO suspension (8 mg ml −1 in DMF:water=9:1 mixture) in a 20-ml glass vial using a micropipette. The vial was then left on a shaker for several hours, typically ~24 h. After that, the samples were rinsed by immersing in DI water for 2–3 days. The DI water was exchanged three times a day. Formation of GO/b-PEI films on substrates Small amount of b-PEI solution (25 wt. % in DI) was applied to the substrate of interest, such as glass slides and filter paper. The substrate was then immersed in a GO suspension (8 mg ml −1 in DMF:water=9:1 mixture) and left on a shaker for several hours, typically ~24 h. For example, film shown in Fig. 4e has been prepared by first applying 1 ml of the b-PEI solution to an 8 cm × 10 cm rectangular area of a filter paper (Whatman, grade no. 3); the substrate was then immersed in 90 ml of the GO suspension and left on a shaker for 24 h. A plastic container with dimensions of 15 cm × 10 cm × 5 cm was used as reaction vessel. After the film formation, samples were rinsed by immersing in DI water for 2–3 days. The DI water was exchanged three times a day. In the case of using a thread as the substrate, the fibre was first immersed in the b-PEI solution for a few seconds and then transferred into a GO suspension. All other procedures are identical. Drying the assembled GO/b-PEI structures After rinsing the samples, freeze-drying was used to get porous foam-like structures. Tightly packed films were obtained by drying the samples in an oven at 80 °C overnight. To prepare structures with intermediate densities, the water in the initial product was exchanged to a solvent with low surface tension such as toluene, hexane and ethanol. After that, the sample was dried in an oven at 80 °C overnight. Sheet resistance measurement of r-GO/b-PEI films GO/b-PEI films were prepared on a filter paper (Whatman, grade no. 3) by the method discussed above. In general, square area of 8 cm × 10 cm was used. The film was dried and then cut into smaller pieces (2 cm × 2 cm), which were reduced in four different ways. (1) HI treatment: sample was immersed in a HI solution (55% in DI) and kept at room temperature overnight. After that, it was rinsed with ethanol until no more iodine residue (identified by the brown colour) was seen coming out. (2) Hydrazine treatment: sample was place in an autoclave with small amount of hydrazine (2% in water) and kept at 80 °C overnight. (3 and 4) Thermal treatment at 220 and 450 °C: sample was placed inside a tube furnace under nitrogen atmosphere. Heating rate was 5 °C min −1 for both cases. The samples were left at the final temperature for 30 min and then taken out. Pure GO films were prepared by placing a PTFE dish containing GO suspension (8 mg ml −1 ) in an 80 °C oven. The dried GO film was cut into 2 cm × 2 cm pieces and reduced the same way as the GO/b-PEI films. Sheet resistant of the reduced films was measured by a Jandel HM21 Portable Four Point Probe Test Meter (cylindrical four point probe head, probe spacing 1 mm). Current was set as 10 mA, and sheet resistance was read out from the metre in Ω □ −1 . Characterization Unless mentioned otherwise, data presented in the manuscript have been collected from samples obtained after reaction time of 24 h. Transmission FT-IR spectra were obtained using a JASCO FT/IR-4200 spectrometer. Measurements were conducted under ambient conditions. Resolution was set to 4 cm −1 with scanning range from 400 to 4,000 cm −1 . Forty-eight scans per samples were recorded, averaged and corrected against the spectrum of pure KBr as background. XRD measurements were performed using a Rigaku RINT2500 with Cu K α radiation ( λ =0.154 nm). SEM images were taken with a JEOL JSM-7001 F4 microscope, using acceleration voltage in the range of 2–15.0 kV. Sample was fixed on a silicon wafer or conductive carbon tape. To minimize charging effects, 5 nm layer of osmium was applied to non-conductive samples before imaging. TGA were performed using a Thermo plus EVO II system (Rigaku). In general, samples were freeze-dried before testing. Measurement was done under nitrogen atmosphere (flow rate of 50 ml h −1 ) with temperature range of 25−500 °C and scan rate of 10 °C min −1 . Composition of b-PEI with the assembled structures was determined by comparing the mass loss between 100 and 500 °C. How to cite this article: Zou, J. & Kim, F. Diffusion-driven layer-by-layer assembly of graphene oxide nanosheets into porous three-dimensional macrostructures. Nat. Commun. 5:5254 doi: 10.1038/ncomms6254 (2014).